Trans- and cis-acting effects ofFirreon epigenetic features of the inactive X chromosome Firre encodes a lncRNA involved in nuclear organization. Here, we show that Firre RNA expressed from the active X chromosome maintains histone H3K27me3 enrichment on the inactive X chromosome (Xi) in somatic cells. This trans-acting effect involves SUZ12, reflecting interactions between Firre RNA and components of the Polycomb repressive complexes. Without Firre RNA, H3K27me3 decreases on the Xi and the Xi-perinucleolar location is disrupted, possibly due to decreased CTCF binding on the Xi. We also observe widespread gene dysregulation, but not on the Xi. These effects are measurably rescued by ectopic expression of mouse or human Firre / FIRRE transgenes, supporting conserved trans-acting roles. We also find that the compact 3D structure of the Xi partly depends on the Firre locus and its RNA. In common lymphoid progenitors and T-cells Firre exerts a cis-acting effect on maintenance of H3K27me3 in a 26 Mb region around the locus, demonstrating cell type-specific trans- and cis-acting roles of this lncRNA. X chromosome inactivation (XCI) is initiated by the long noncoding RNA (lncRNA) Xist , which becomes highly expressed on one allele, and coats the future inactive X chromosome (Xi) in cis [1] , [2] , [3] , [4] , [5] . Specific proteins that include components of the Polycomb repressive complexes PRC1 and PRC2 are recruited by Xist RNA to mediate serial layers of epigenetic modifications, resulting in gene silencing and heterochromatin formation [2] , [6] , [7] . Epigenetic hallmarks of the Xi include multiple repressive histone modifications such as ubiquitination of histone H2A at lysine 119 (H2AK119ubi), tri-methylation of histone H3 at lysine 27 (H3K27me3), and enrichment in the histone variant macroH2A1 [8] . Additional layers of control ensure stability of the silent state of the Xi, including DNA methylation of promoter-containing CpG islands, a shift to late replication, and spatial reorganization of the Xi within the nucleus [9] , [10] . The Xi appears as the heteropycnotic Barr body usually located close to either the nuclear lamina or the periphery of the nucleolus [11] , [12] , [13] , [14] , [15] . These two locations are preferred sites of heterochromatin, not only for the Xi but also for other repressed regions of the genome, suggesting that their proximity helps maintain silent chromatin [11] , [16] . In particular, the perinucleolar space has a primary function in replication and maintenance of repressive chromatin state [17] , [18] . The factors and mechanisms that facilitate association of heterochromatic regions including the Xi to specific nuclear compartments such as the lamina or the nucleolus remain elusive. Xist RNA interaction with the lamin B receptor (LBR) has been proposed as a critical factor that recruits the Xi to the lamina and facilitates silencing [19] . Our previous studies suggest that perinucleolar positioning of the Xi may be facilitated by the lncRNA Firre [20] . The Firre locus comprises conserved tandem repeats that bind CTCF specifically on the Xi but not on the Xa (active X chromosome) [20] , [21] , [22] . Despite sequence divergence between species, the conserved nature of the repeat locus suggests important roles in mammals [21] . Firre RNA is usually confined to the nucleus where it interacts with the nuclear matrix protein hnRNPU [23] , [24] . Multiple transcript isoforms including circular RNAs, further complicate an understanding of the roles of Firre in different cell types [25] . On the Xi the Firre locus contacts the Dxz4 locus that also binds CTCF only on the Xi [26] , [27] , [28] . Dxz4 is necessary for the formation of the bipartite structure of the Xi [27] , [29] , [30] , [31] . The Firre locus also interacts with several autosomal regions, consistent with a widespread role in nuclear architecture [23] , [32] . A Firre knockout (KO) mouse model is viable, but results in cell-type-specific defects in hematopoiesis that impact common lymphoid progenitors (CLPs) [32] , [33] . Importantly, these defects are rescued by ectopic expression of Firre from an autosomal location, thus defining a trans-acting role for Firre [32] , [33] . KO mice show organ-specific dysregulation of autosomal genes, consistent with physiological defects in distinct phases of hematopoiesis [32] . Here, we investigate the role of Firre in maintenance of heterochromatin, gene expression, and 3D structure of the Xi by engineering allele-specific deletions of the Firre locus and by Firre knockdown (KD) in mouse cell lines and tissues. Depletion of Firre RNA reveals important roles in H3K27me3 enrichment on the Xi and in location of the Xi within the nucleus as shown by immunostaining, ChIP-seq, and CUT&RUN. Gene expression is disrupted, as is the 3D structure of the Xi as shown by RNA-seq, ATAC-seq, and Hi-C. Our results are supported by rescue experiments using cDNA transgenes. We demonstrate both trans- and cis-acting roles of Firre RNA and its locus, with evidence of cell-type-specific effects in cell lines and in vivo. Firre and CrossFirre are transcribed from the Xa Allele-specific CRISPR/Cas9 editing of the Firre region was done in Patski cells, in which skewed XCI and species-specific SNPs allowed us to design guides to target the Xi from BL6 or the Xa from Mus spretus ( spretus ) (Supplementary Data 1 ). We isolated single-cell clones with either a ~160 kb deletion of Firre on the Xa (Δ Firre Xa ), a ~160 kb deletion of Firre on the Xi (Δ Firre Xi ), or a ~160 kb inversion of Firre on the Xi (Inv Firre Xi ) (Fig. 1a ). Deletion of the Firre locus on the Xa resulted in undetectable Firre expression by RT-PCR, while deletion on the Xi caused no change (Fig. 1a, b , Supplementary Data 2 ). Allele-specific RNA-seq analysis confirmed the absence of Firre transcripts from either Xa or Xi in Δ Firre Xa , while control loci ( Dxz4 , Xist ) showed no change (Supplementary Data 3 ). Fig. 1: Firre and CrossFirre are expressed from the Xa. a Genomic location of Firre and CrossFirre ( Gm35612 ) on the mouse X chromosome (UCSC mm10 build 38 browser tracks). Note that Firre has multiple alternative transcripts. The locations of the CRISPR guide RNAs used to edit the locus (cut), and of the RT-PCR primer pairs to specifically detect Firre expression (F/R), strand-specific expression of CrossFirre (F1/R1), or strand-specific expression in a region of overlap between Firre and CrossFirre (F2/R2) are indicated. b RT-PCR analysis using the F/R primer pair detects Firre expression in WT, Δ Firre Xi , and Inv Firre Xi , but not in Δ Firre Xa . Firre expression was measured in n = 3 biologically independent samples per cell type. c Sanger sequencing analyses of a CrossFirre region (F1/R1) and of a region of overlap between Firre and CrossFirre (F2/R2) confirm heterozygosity of SNPs (BL6 on the Xi and spretus on the Xa) in each region assayed. Genomic DNA (gDNA) shows heterozygosity at the SNPs, while cDNA only shows expression from the spretus SNP (Xa). d Strand-specific analysis of CrossFirre and Firre was done using reverse transcription using either random primers, or F1, R1, F2, R2 primers, followed by PCR using F1/R1 or F2/R2 primer pairs. Firre and CrossFirre expression was measured in n = 3 biologically independent samples per cell type. Source data are provided as a Source Data file. Full size image Our Δ Firre Xa deletion includes the antisense transcript CrossFirre that partially overlaps Firre (Fig. 1a ; Supplementary Fig. 1a ) [34] . Note that, in contrast to Δ Firre Xa , previously constructed Firre deletions in mouse ES cells and in a KO mouse do not include all of CrossFirre [32] , [35] . To test CrossFirre expression in edited Patski cells, we processed strand-specific RT-PCR using primers (F1/R1) that flank a 231 bp region in the middle of CrossFirre with no Firre overlap, and primers (F2/R2) that flank a 203 bp region overlapping the 3’ end of Firre (Fig. 1a ). For the non-overlapped region, forward CrossFirre transcripts containing only SNPs from the Xa ( spretus ), were present in WT (wild-type), Δ Firre Xi , and Inv Firre Xi , but absent in Δ Firre Xa (Fig. 1c, d ). For the overlapped region, transcripts from both directions ( CrossFirre and Firre ), again containing only SNPs from the Xa ( spretus ), were present in WT, Δ Firre Xi , and Inv Firre Xi , but absent in Δ Firre Xa (Fig. 1d ). We found no evidence of miRNAs in the Firre/CrossFirre region using miRNA-seq in WT or Δ Firre Xa , suggesting that the loci function independently of the small RNA pathway (Supplementary Data 4 ). We conclude that Firre and CrossFirre are both transcribed from the Xa in Patski cells. Note that Firre was originally identified as a gene that escapes XCI in human and mouse [20] , [23] , [28] . However, our current results and those reported in Firre KO mouse ES cells and in KO mice clearly show that Firre is predominantly expressed from the Xa in fibroblasts [32] , [35] . Firre acts in trans to maintain PRC2 and H3K27me3 on the Xi To determine whether any of the allelic alterations constructed, Δ Firre Xa , Δ Firre Xi , and Inv Firre Xi , influences epigenetic marks on the Xi, immunostainings for H3K27me3, H2AK119ubi, and macroH2A.1 were done in combination with Xist RNA-FISH to locate the Xi. The majority of nuclei (95 ± 3%) had one Xist cloud in all edited cell lines, indicating no disruption of Xist RNA coating (Fig. 2a ). A strong H3K27me3 immunostaining cluster was observed on the Xi in 83 ± 2% of WT nuclei as expected. In contrast, only 9 ± 2% of nuclei with a H3K27me3 cluster were observed in Δ Firre Xa , with most nuclei appearing uniformly mottled throughout (Fig. 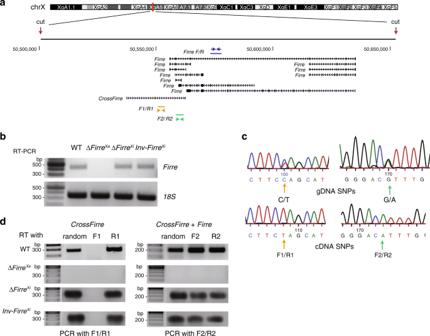Fig. 1:FirreandCrossFirreare expressed from the Xa. aGenomic location ofFirreandCrossFirre(Gm35612) on the mouse X chromosome (UCSC mm10 build 38 browser tracks). Note thatFirrehas multiple alternative transcripts. The locations of the CRISPR guide RNAs used to edit the locus (cut), and of the RT-PCR primer pairs to specifically detectFirreexpression (F/R), strand-specific expression ofCrossFirre(F1/R1), or strand-specific expression in a region of overlap betweenFirreandCrossFirre(F2/R2) are indicated.bRT-PCR analysis using the F/R primer pair detectsFirreexpression in WT, ΔFirreXi, and InvFirreXi, but not in ΔFirreXa.Firreexpression was measured inn= 3 biologically independent samples per cell type.cSanger sequencing analyses of aCrossFirreregion (F1/R1) and of a region of overlap betweenFirreandCrossFirre(F2/R2) confirm heterozygosity of SNPs (BL6 on the Xi andspretuson the Xa) in each region assayed. Genomic DNA (gDNA) shows heterozygosity at the SNPs, while cDNA only shows expression from thespretusSNP (Xa).dStrand-specific analysis ofCrossFirreandFirrewas done using reverse transcription using either random primers, or F1, R1, F2, R2 primers, followed by PCR using F1/R1 or F2/R2 primer pairs.FirreandCrossFirreexpression was measured inn= 3 biologically independent samples per cell type. Source data are provided as a Source Data file. 2b ; Table 1 ). There was no evidence of a complete loss of H3K27me3 over the Xi, which would have appeared as a “hole” with complete absence of immunostaining. H3K27me3 level throughout Δ Firre Xa and WT nuclei was measured in regions outside the Xi using ImageJ to quantify fluorescence intensity by normalization to DNA or to histone panH4 [36] . No significant difference was detected in regions outside the Xi between Δ Firre Xa and WT, but subtle or local changes undetectable by immunostaining cannot be excluded (Supplementary Fig. 2a, b ). Δ Firre Xi and Inv Firre Xi nuclei retained a strong H3K27me3 cluster on the Xi, consistent with retention of Firre RNA in these cells (Fig. 2b ). Two other histone modifications known to be associated with XCI, H2AK119ubi and macroH2A.1, showed no changes in Δ Firre Xa nuclei (Fig. 2c ). Fig. 2: Firre RNA acts in trans to maintain H3K27me3 on the Xi. a – c A total of >300 Patski nuclei were scored per cell type over 3 independent experiments; significance was determined by one-sided Fisher exact test; bar plots are presented as mean values ± SEM; scale bars represent 10 µm. a Examples of nuclei after Xist RNA-FISH (green) and Hoechst 33342 staining (blue). The bar plot shows no significant differences among cell lines. b Examples of nuclei after H3K27me3 immunostaining (red) and Hoechst 33342 staining (blue). The bar plot shows significantly fewer nuclei with a H3K27me3 cluster in Δ Firre Xa versus WT ( p value = 4.63688e-94), but no change in Δ Firre Xi nor Inv Firre Xi . c Examples of nuclei after macroH2A.1 or H2AK119ubi (red) immunostaining and Hoechst 33342 staining (blue). The bar plots show no significant differences between cell types. d Profiles of H3K27me3 ChIP-seq reads along the Xi in WT (blue), Δ Firre Xa (red), and log 2 ratio Δ Firre Xa /WT (green). Box plots (log 2 ) of H3K27me3 ChIP-seq reads in 100 bp Xi bins show a significantly lower median in Δ Firre Xa (red) versus WT (blue) (Wilcoxon test: p value = 2.2e-16). The boxes demarcate the interquartile range (IQR) with median; whiskers ±1.5 times the IQR; outliers plotted as points. e Density histograms of the distribution of allelic proportions (Xa/(Xa+Xi)) of H3K27me3 peaks show a shift for the X chromosomes due to lower H3K27me3 on the Xi in Δ Firre Xa (red) compared to WT (blue) (Wilcoxon test: −log10P = inf). f Heatmaps of H3K27me3 ChIP-seq reads 3 kb around transcription start sites (TSS) of genes on the Xi in Δ Firre Xa versus WT. g . Metagene plots of average H3K27me3 occupancy at X-linked genes ((TSS to termination site (TES), not at scale)) in Δ Firre Xa (Xi red Xa pink) versus WT (Xi blue, Xa purple). h Density histograms of the distribution of allelic proportions (Xa/(Xa+Xi)) of SUZ12 peaks show a shift for the X chromosomes due to lower SUZ12 on the Xi in Δ Firre Xa (red) versus WT (blue) (Wilcoxon test: −log10P = 20.98). i Genome tracks demonstrating interactions between hnRNPK, EZH2, and SUZ12 with Firre RNA based on RIP-seq data in trophoblast and embryo stem cells [39] , [40] . Full size image Table 1 Percentages of nuclei with a H3K27me3 cluster on the Xi. Full size table Next, allele-specific profiles of H3K27me3 were generated by ChIP-seq, which demonstrated a chromosome-wide decrease on the Xi in Δ Firre Xa (Fig. 2d ). The loss of H3K27me3 in mutant cells was quantified by counting unique reads mapped to the Xa, Xi, and autosomes. In WT the Xi/Xa read ratio was 2.45, reflecting the characteristic H3K27me3 enrichment on the Xi. In contrast, this ratio was only 1.60 in Δ Firre Xa , representing a significant decrease on the Xi (Fig. 2d ). The BL6/ spretus read ratios for autosomes in WT and Δ Firre Xa remained similar, 1.04 and 1.14, respectively. The 34% percent decrease in the level of H3K27me3 on the Xi as measured by ChIP-seq is lower than that measured by immunostaining (89%), which is expected based on known differences between methodologies. While immunostaining captures condensation of the Xi and thus results in many nuclei with a visible H3K27me3 cluster, ChIP-seq reveals uneven distribution of H3K27me3 along the Xi and thus an apparently lesser enrichment [37] . In fact, the 34% change in H3K27me3 we measured by ChIP-seq in Δ Firre Xa versus WT is similar to that reported between undifferentiated and differentiated mouse ES cells, in which the onset of XCI causes only a 40% increase in H3K27me3 level as measured by ChIP-seq, while over 90% of nuclei acquire a visible H3K27me3 cluster, as determined by immunostaining [37] . Next, we calculated allelic proportions of SNP read coverage for each H3K27me3 peak covered by at least five SNP reads. In both WT and Δ Firre Xa the distribution of allelic proportions ( spretus /( spretus + BL6)) for the autosomes centered close to the anticipated 0.5, reflecting a similar enrichment between alleles (Fig. 2e ). In contrast, the distribution of allelic proportions for the X chromosomes (Xa/(Xa + Xi)) centered at ~0.35 in WT, consistent with H3K27me3 enrichment on the Xi, but was markedly shifted to higher values (~0.5) in Δ Firre Xa , supporting the 34% decrease in H3K27me3 on the Xi (Fig. 2e ). Heatmaps and metagene plots of allelic ChIP-seq data further demonstrate a dramatic loss of H3K27me3 around the transcription start site and throughout the body of X-linked genes in mutant cells (Fig. 2f, g ). LINE and SINE repeats also show lower H3K27me3 on the Xi in Δ Firre Xa (Supplementary Fig. 2c ). Finally, we confirmed a decrease in H3K27me3 in Δ Firre Xa using CUT&RUN in a separate study [38] . Next, we investigated SUZ12, a subunit of the PRC2 complex, using CUT&RUN, which showed a decrease on the Xi in Δ Firre Xa . Again, the distribution of allelic proportions (Xa/(Xa+Xi)) for each SUZ12 peak showed a pronounced shift toward higher values (~0.75) for the X chromosomes in Δ Firre Xa versus WT, while allelic proportions for the autosomes (0.5) did not change (Fig. 2h ). Reanalysis of published datasets of RNA/protein interactions in mouse cells confirmed Firre RNA interactions with PRC components. Analysis of RIP-seq data showed Firre RNA interactions with two components of PRC2, EZH2 and SUZ12, and with hnRNPK, a protein that recruits the noncanonical PCGF3/5-PRC1 (Fig. 2i ; Supplementary Data 5 ) [39] , [40] . Analysis of data obtained by CLIP-seq and PAR-CLIP, two UV-crosslinking-based methods for highly accurate mapping of RNA-protein interactions, confirmed Firre RNA interactions with EZH2 and detected interactions with JARID2 and RBFOX2, two proteins known to help recruit PRC2 to chromatin, and with CBX7, a component of the canonical PRC1 complex implicated in H3K27me3 deposition [41] , [42] , [43] , [44] , [45] (Supplementary Data 5 ). We conclude that Firre RNA transcribed from the Xa specifically helps target PRC1 and PRC2 complexes to the Xi for maintenance of H3K27me3, consistent with a trans-acting effect in Patski cells. In support we find that several proteins implicated in the PRC complexes are Firre RNA interactors. Dose-dependent and cell-type-specific effects of Firre To quantify the effects of Firre , we knocked it down in a dose-dependent manner using shRNA and siRNA treatments of an independent Patski isolate to achieve KD levels ranging from 43, 28, and 10% of WT. This caused a parallel reduction in percentages of nuclei with a H3K27me3 cluster to 33%, 27%, and 15%, respectively, versus 83% in WT ( p < 0.0001) (Fig. 3a ; Table 1 ). Importantly, this reveals a dose-dependent effect of Firre RNA on H3K27me3 enrichment on the Xi (Fig. 3a ). Concomitantly, a dose-dependent increase in CrossFirre RNA inversely correlates to the amount of Firre RNA, consistent with Firre repressing the antisense transcript (Fig. 3b ). Fig. 3: Dose-dependent effects of Firre RNA on H3K27me3 on the Xi in cell lines and in vivo. a Percentage of nuclei with a H3K27me3 cluster after KD in Patski cells relative to Firre expression level measured by qRT-PCR in n = 3 biologically independent samples. Data presented as mean values ± SEM. b The level of CrossFirre expression is inversely related to that of Firre after Firre KD. Expression measured by qRT-PCR in n = 3 biologically independent samples. Data presented as mean values ± SEM. c, d A total of >300 Patski nuclei were scored per cell type over three independent experiments; significance was determined by one-sided Fisher exact test; bar plots are presented as mean values ± SEM; scale bars represent 10 µm. c Bar plots show significantly fewer H3K27me3 clusters after Firre KD in nuclei from three primary MEFs compared to mock treatment ( p value = 2.89075e-12, 1.41519e-32, and 8.95838e-10, respectively). Primary MEFs were derived from a (BL6 × spretus ) embryo with a spretus Xi, and from embryos either (BL6 × spretus ) or (BL6 × castaneus ) with random XCI (Table1). d Bar plots show a lower (but not significantly) percentage of H3K27me3 cluster in nuclei from MEFs derived from Firre +/− and Firre −/− KO embryos than in controls ( p value = 0.0774 and 0.0567, respectively). No significant differences were found in brain, liver, and kidney from Firre KO mice compared to WT ( p value = 0.9127, 0.8796, and 0.762, respectively). e Profiles of H3K27me3 ChIP-seq reads along the X chromosomes from CLPs and CD8 + T cells from WT (blue), Firre −/− (red), and log 2 ratio Firre −/− /WT (green) show a significant decrease covering ~26 Mb around the Firre locus in mutant CLPs, and to a lesser extent CD8 + T cells (Supplementary Data 6 ). f Heatmaps of H3K27me3 ChIP-seq reads located 3 kb around the transcription start sites (TSS) of X-linked genes that map within the 26 Mb region around Firre in WT and Firre −/− CLPs and CD8 + T cells. Full size image A separate KD to deplete Firre RNA to 33% of WT in primary mouse embryonic fibroblasts (MEFs) independently derived from a BL6 × spretus F1 embryo with random XCI significantly decreased the percentage of nuclei with a H3K27me3 cluster to 43%, versus 79% in controls ( p < 10 −4 ) (Fig. 3c ; Table 1 ). To exclude species-specific effects, we tested MEFs from a BL6 × spretus F1 embryo with an XCI pattern opposite to that in Patski cells (i.e., the Xi is from spretus ), and MEFs from a BL6 × castaneus F1 embryo. After KD in these lines Firre RNA level was lowered to 21 and 15% of WT, causing a significant reduction to 45 and 47% of nuclei with a H3K27me3 cluster, compared to 80 and 78% in controls, respectively ( p < 10 −4 ) (Fig. 3c ; Supplementary Fig. 2d ; Table 1 ). No significant change in CrossFirre was found in those lines (Supplementary Fig. 2e ). We then examined cells and tissues from a Firre KO mouse model [32] , [33] . MEFs from heterozygous ( Firre +/− ) and homozygous ( Firre −/− ) KO female embryos showed a modest reduction to 43 and 41% of nuclei with a H3K27me3 cluster, respectively, compared to 58% in a control littermate ( Firre +/+ ) (Fig. 3d ; Table 1 ). H3K27me3 immunostaining in liver, kidney, and brain sections derived from Firre −/− female mice showed no significant decrease in nuclei with a cluster (Fig. 3d ; Table 1 ). Next, we performed H3K27me3 ChIP-seq analysis of sorted CLPs and CD8 + T cells derived from Firre −/− KO female mice. Surprisingly, we found a striking loss of H3K27me3 in a ~26 Mb (ChrX: 36–62 Mb) region centered around the Firre locus, together with a slight decrease across the entire X chromosome, but not the autosomes (Fig. 3e , Supplementary Fig. 3a, b ). Heatmaps of control and Firre −/− KO CLPs and CD8 + T cells showed a loss of H3K27me3 around the transcription start site of genes located within this 26 Mb region (Fig. 3f , Supplementary Data 6 ). Although we assume that this local loss of H3K27me3 affects the Xi and not the Xa, allelic analysis was not possible since KO mice are homozygous BL6. The 26 Mb region around Firre contains 266 curated genes, 15 involved in immunity (e.g., Nkap, Sash3, Atp11c , Sh2d1a , Elf4 [46] , [47] , [48] ), and 15 potentially exhibiting haploinsufficiency effects in human (e.g., GPC3 [49] ) (Supplementary Data 6 ). However, no specific expression changes have been reported for any of these genes in CLPs from KO mice [33] . In summary, we found a dose-dependent effect of Firre RNA in maintenance of H3K27me3 on the Xi in several types of fibroblasts. Lack of detectable changes in three tissues from Firre KO mice suggests that the role of Firre may be cell-type- and tissue-specific, as proposed for other lncRNAs [50] . Consistent with the role of Firre in hematopoiesis, local changes were observed in CLPs and CD8 + T cells around the Firre locus, revealing a cell-type-specific role in cis-maintenance of H3K27me3 [33] . Rescue of H3K27me3 on the Xi by Firre/FIRRE cDNA transgenes To confirm a causative role of Firre RNA on H3K27me3 enrichment on the Xi, Δ Firre Xa cells were transfected with a mouse Firre cDNA transgene that lacks the first five 5’ exons of Firre and is expressed from a CMV promoter (Supplementary Fig. 1b ). By RNA-seq Firre expression was restored to a near-normal level after transfection. Ectopic expression of the mouse cDNA in Δ Firre Xa+mtransgene cells rescued the presence of a H3K27me3 cluster from 9 to 38% of nuclei, supporting a trans-acting role (Fig. 4a, b , Table 1 ). This partial rescue is not readily explained by heterogeneous transgene levels among cells, since a cloned transgenic line with stable high Firre expression rescued to a similar level (34%). Firre RNA-FISH in this clone showed association of the lncRNA to the Xist cloud in 15% of cells, consistent with partial rescue (Fig. 4c ). Incomplete rescue is likely due to the partial cDNA transgene that may lack functional RNA motifs, isoforms, and regulatory elements (Supplementary Fig. 1b ). Interestingly, we also observed partial rescue after ectopic expression of a human FIRRE cDNA in Δ Firre Xa+htransgene cells (Fig. 4a, b ; Table 1 ). Next, we examined Firre +/− and Firre −/− MEFs from KO mice with an ectopic doxycycline (DOX)-inducible plasmid copy of a complete Firre cDNA integrated in the genome. After Firre expression induction (10–20 fold) a strong increase to 91 and 83% of nuclei with a H3K27me3 cluster was found compared to 43 and 41% in noninduced KO cells, respectively (Fig. 4d ; Table 1 ). Fig. 4: Ectopic expression of Firre/FIRRE RNA partially restore H3K27me3 on the Xi. a Examples of nuclei after H3K27me3 immunostaining (red) and Hoechst 33342 staining (blue) in WT, Δ Firre Xa , and Δ Firre Xa transfected with a mouse Firre transgene (Δ Firre Xa+mtransgene ) or a human FIRRE transgene (Δ Firre Xa+htransgene ). b The bar plot shows a significantly higher percentage of nuclei with a H3K27me3 cluster in cells with a mouse or human Firre/FIRRE transgene, compared to Δ Firre Xa ( p value = 2.8075e-16 and 0.0000134599, respectively). c Examples of nuclei after RNA-FISH for Xist (green) and Firre (red) in a Δ Firre Xa+mtransgene cell clone with high expression of the mouse transgene. The upper two nuclei show association between Firre and Xist signals (seen in 15% of nuclei), and the lower nuclei, lack of association. d The bar plot shows the percentage of nuclei with a H3K27me3 cluster in MEFs derived from Firre +/− and Firre −/− females that harbor a doxycycline (Dox) inducible transgene ( Firre +/− tg;rtTA; -Dox; Firre +/− tg;rtTA; +Dox; Firre −/− tg;rtTA; -Dox; Firre −/− tg;rtTA; +Dox), compared to WT and mutants. The percentage of nuclei with a H3K27me3 cluster increases significantly in Firre +/− tg;rtTA and Firre −/− tg;rtTA MEFs after addition of doxycycline (Dox+) (p value=4.31567e-30 and 3.51193e-20, respectively). A total of >300 nuclei scored for the presence of a H3K27me3 cluster ( a , b, d ), or for Xist and Firre RNA-FISH signals ( c ) per cell type over three independent experiments; significance was determined by one-sided Fisher exact test; bar plots are presented as mean values ± SEM; scale bars represent 10 µm. Full size image We conclude that loss of H3K27me3 on the Xi in mutant cells is rescuable by a cDNA transgene, supporting Firre trans-acting role. Surprisingly, a human FIRRE transgene can also rescue to some extent, suggesting functional compatibility between species despite sequence divergence. Results of induction of a transgene in the mouse KO model further support a dose-dependent trans-effect of Firre RNA on H3K27me3 enrichment on the Xi. Firre acts in trans to maintain nuclear location of the Xi We next examined the effects of allelic Firre mutations on the Xi location relative to the nucleolus and lamina. In WT, Δ Firre Xi , and Inv Firre Xi H3K27me3 and nucleophosmin (NPM1) immunostaining was used to locate the Xi and the nucleoli, respectively (Fig. 5a ). Since the H3K27me3 cluster is compromised in Δ Firre Xa , Xist RNA-FISH was applied in combination with NPM1 immunostaining. The Xi location was scored in WT nuclei as adjacent to the nuclear periphery (70%), the nucleolus surface (50%), or neither (8%) (Fig. 5b ). Note that in 28% of nuclei the Xi was close to both the periphery and the nucleolus. Loss of Firre RNA in Δ Firre Xa caused significant reductions in Xi-nuclear periphery and Xi-nucleolus associations to 20 and 22% of nuclei, respectively ( p < 0.0001) (Fig. 5b ). Importantly, ectopic expression of a cDNA transgene in Δ Firre Xa+mtransgene significantly (but not completely) rescued these associations (Fig. 5b ). Deletion or inversion of Firre on the Xi did not alter its location (Fig. 5a, b ). In primary MEFs independently derived from a BL6 × spretus F1 mouse with random XCI Firre KD also caused a decrease in Xi-nuclear periphery and Xi-nucleolus associations (Fig. 5c ). Fig. 5: Firre RNA acts in trans to maintain Xi location. a – c A total of >300 nuclei per cell type over 3 independent experiments were scored for the location of the Xi marked by a H3K27me3 cluster or an Xist cloud relative to the nuclear periphery or the nucleolus; significance was determined by one-sided Fisher exact test; bar plots are presented as mean values ± SEM; scale bars represent 10 µm. a Examples of nuclei after H3K27me3 immunostaining (red) to locate the Xi in WT, Δ Firre Xi , and Inv Firre Xi , or Xist RNA-FISH (red) to locate the Xi in Δ Firre Xa since there is no H3K27me3 cluster in these nuclei. Nuclei were also immunostained for NPM1 (green) to locate the nucleolus. b Bar plots show a significant decrease in periphery- and nucleolus association of the Xi in Δ Firre Xa compared to WT ( p value = 3.95632e-40 and 3.75497e-14, respectively), but no significant changes in Δ Firre Xi and Inv Firre Xi ( p value = 0.6968). Ectopic expression of a mouse transgene in Δ Firre Xa+mtransgene partly rescues the Xi location to 41% at the periphery and 34% at the nucleolus ( p value = 6.62701e-10 and 0.000265481, respectively). c Bar plots show a significant decrease in periphery- and nucleolus association of the Xi after Firre KD in primary MEFs derived from an F1 embryo (BL6 × spretus ) ( p value = 1.13757e-09 and 0.0000634923, respectively). d Density histograms of the distribution of allelic proportions (Xa/(Xa + Xi)) of CTCF peaks show a shift in the distribution for the X chromosomes due to a decrease in CTCF on the Xi in Δ Firre Xa (red) compared to WT (blue). In Δ Firre Xa+mtransgene (brown) this distribution becomes binomial due to partial restoration of CTCF on the Xi. e Plots of Xi-associated (common +Xi-specific) CTCF peak density (counts binned within 100 kb windows) along the Xi for WT (blue) and Δ Firre Xa (red). To account for differences in the number of SNP-covered peaks due to sequencing depth, the binned counts are scaled by a factor obtained from the between-sample ratios of autosomal diploid SNP-covered peaks. Full size image CTCF has been implicated in nucleolus association of genomic regions, and we have previously shown that Ctcf KD reduces Xi-nucleolus associations in Patski cells [20] , [51] . Here, we profiled allelic CTCF binding by CUT&RUN, which demonstrated a loss of CTCF binding on the Xi in Δ Firre Xa (Fig. 5d ). The distribution of allelic proportions (Xa/(Xa + Xi)) for CTCF peaks on the X chromosomes showed a pronounced shift toward higher values (~0.85) in Δ Firre Xa compared to WT (~0.65), while allelic proportions ( spretus /( spretus + BL6)) for the autosomes were close to the anticipated 0.5 (Fig. 5d ). Thus, while there is less CTCF binding on the Xi versus Xa in WT as expected, CTCF binding is even lower in Δ Firre Xa (Fig. 5e ). In Δ Firre Xa+mtransgene the distribution of allelic proportions for the X chromosomes becomes binomial, indicating partial restoration of CTCF on the Xi (Fig. 5d ). Taken together, our results show that Firre RNA transcribed from the Xa or from an ectopic cDNA transgene can influence in trans the Xi location within the nucleus. Our results further suggest a potential cooperation between Firre RNA and CTCF in maintenance of Xi location. Loss of Firre affects gene expression in Patski cells Next, we examined changes in total gene expression (autosomal and X-linked genes without allele discrimination) in Δ Firre Xa . About 11 and 14% of genes with expression ≥1TPM in at least one condition were upregulated and downregulated in Δ Firre Xa versus WT, respectively, (Supplementary Data 7 and 8 ). A large proportion (46 and 40%, respectively) of dysregulated genes were rescued in Δ Firre Xa+mtransgene (Fig. 6a, b , Supplementary Fig. 4a , Supplementary Data 7 ). To rule out effects of aneuploidy between cell lines results were confirmed for genes located on diploid chromosomes in WT and Δ Firre Xa (Supplementary Fig. 4b , Supplementary Data 9 ). GO analysis show that the top 20 GO terms for genes upregulated in Δ Firre Xa and rescued in Δ Firre Xa+mtransgene are related to cell cycle, DNA replication, chromosome segregation, and immune cell function, while downregulated genes are implicated in development, differentiation, and metabolism (Fig. 6a, b ; Supplementary Data 10 ). In human HEK293 cells FIRRE RNA KD resulted in dose-dependent cell death, consistent with a role in cell growth and survival (Supplementary Fig. 4c ). Fig. 6: Loss of Firre RNA affects gene expression. a Upregulated genes in Δ Firre Xa and Gene Ontology (GO) term enrichment. The Venn diagram shows the number of upregulated genes in Δ Firre Xa versus WT, and in Δ Firre Xa versus Δ Firre Xa+mtransgene , with the overlapping gene set representing upregulated genes in Δ Firre Xa that are rescued by transgene expression. The scatter plot shows dysregulated genes in Δ Firre Xa versus WT (grey), with genes rescued by reduced expression in Δ Firre Xa+mtransgene versus Δ Firre Xa (more than 2-fold; p value < 0.05 by the Wald test) highlighted in orange. The top 20 GO terms of overlapping upregulated genes in Δ Firre Xa versus WT, which are rescued in Δ Firre Xa+mtransgene are listed. The X -axis indicates the FDR (−log10). b Downregulated genes in Δ Firre Xa and Gene Ontology (GO) term enrichment. The Venn diagram shows the number of downregulated genes in Δ Firre Xa versus WT, and in Δ Firre Xa versus Δ Firre Xa+mtransgene , the overlapping gene set representing downregulated genes in Δ Firre Xa that are rescued by transgene expression. The scatter plot shows dysregulated genes in Δ Firre Xa versus WT (gray), with genes rescued by increased expression in Δ Firre Xa+mtransgene versus Δ Firre Xa (more than 2-fold; p value <0.05 by the Wald test) highlighted in blue. The top 20 GO terms of overlapping downregulated genes in Δ Firre Xa versus WT, which are rescued in Δ Firre Xa+mtransgene are listed. 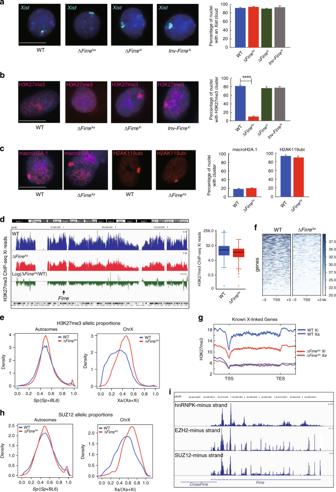Fig. 2:FirreRNA acts in trans to maintain H3K27me3 on the Xi. a–cA total of >300 Patski nuclei were scored per cell type over 3 independent experiments; significance was determined by one-sided Fisher exact test; bar plots are presented as mean values ± SEM; scale bars represent 10 µm.aExamples of nuclei afterXistRNA-FISH (green) and Hoechst 33342 staining (blue). The bar plot shows no significant differences among cell lines.bExamples of nuclei after H3K27me3 immunostaining (red) and Hoechst 33342 staining (blue). The bar plot shows significantly fewer nuclei with a H3K27me3 cluster in ΔFirreXaversus WT (pvalue = 4.63688e-94), but no change in ΔFirreXinor InvFirreXi.cExamples of nuclei after macroH2A.1 or H2AK119ubi (red) immunostaining and Hoechst 33342 staining (blue). The bar plots show no significant differences between cell types.dProfiles of H3K27me3 ChIP-seq reads along the Xi in WT (blue), ΔFirreXa(red), and log2ratio ΔFirreXa/WT (green). Box plots (log2) of H3K27me3 ChIP-seq reads in 100 bp Xi bins show a significantly lower median in ΔFirreXa(red) versus WT (blue) (Wilcoxon test:pvalue = 2.2e-16). The boxes demarcate the interquartile range (IQR) with median; whiskers ±1.5 times the IQR; outliers plotted as points.eDensity histograms of the distribution of allelic proportions (Xa/(Xa+Xi)) of H3K27me3 peaks show a shift for the X chromosomes due to lower H3K27me3 on the Xi in ΔFirreXa(red) compared to WT (blue) (Wilcoxon test: −log10P = inf).fHeatmaps of H3K27me3 ChIP-seq reads 3 kb around transcription start sites (TSS) of genes on the Xi in ΔFirreXaversus WT.g. Metagene plots of average H3K27me3 occupancy at X-linked genes ((TSS to termination site (TES), not at scale)) in ΔFirreXa(Xi red Xa pink) versus WT (Xi blue, Xa purple).hDensity histograms of the distribution of allelic proportions (Xa/(Xa+Xi)) of SUZ12 peaks show a shift for the X chromosomes due to lower SUZ12 on the Xi in ΔFirreXa(red) versus WT (blue) (Wilcoxon test: −log10P = 20.98).iGenome tracks demonstrating interactions between hnRNPK, EZH2, and SUZ12 withFirreRNA based on RIP-seq data in trophoblast and embryo stem cells39,40. The X -axis indicates the FDR (−log10). c Xi-expression fold changes for genes that are subject to or escape XCI between Δ Firre Xa and WT. Upregulated genes are in red and downregulated genes in green. To note, one upregulated gene and one gene subject to XCI are in gray, as they showed more than 2-fold change in expression but with a p value >0.05 by the Wald test in Δ Firre Xa versus WT. Genes are ordered from centromere to telomere along the Xi. Full size image To determine whether gene expression was disrupted on the Xi upon loss of Firre RNA we evaluated allelic gene expression. Only 6/352 genes known to be subject to XCI showed >2-fold upregulation in Δ Firre Xa , suggesting minor Xi reactivation (Fig. 6c , Supplementary Data 3 and 7 ). Four of the reactivated genes were located at the telomeric end of the Xi where higher accessibility and decreased contact density were observed by ATAC-seq and Hi-C (see below). Although their number is small and we cannot rule out a chance occurrence, more genes known to escape XCI were dysregulated (10–14%) from the Xi than genes subject to XCI (2–3%) (Fig. 6c , Supplementary Fig. 4d , Supplementary Data 7 ). A majority of dysregulated X-linked genes (67%) were rescued in Δ Firre Xa+mtransgene (Supplementary Fig. 4e , Supplementary Data 3 and 7 ). Metagene plots of H3K27me3 along autosomal and X-linked genes grouped based on their expression changes in Δ Firre Xa , together with profiles of individual genes showed a small increase in H3K27me3 for downregulated genes, and very little or no change for upregulated or unchanged genes (Supplementary Fig. 5a, b ). Note that 90% of dysregulated genes have no H3K27me3 enrichment in either WT or Δ Firre Xa . Additional CUT&RUN analyses of two active epigenetic marks, H3K36me3 and H3K4me3, showed no significant changes on the Xi in Δ Firre Xa , consistent with little Xi reactivation (Supplementary Fig. 5c, d ) Thus, the loss of Firre RNA causes widespread changes in gene expression in large part rescued by a cDNA transgene. Very little reactivation and few changes in escape genes occur on the Xi despite the observed loss of H3K27me3, consistent with this epigenetic mark representing only one layer of XCI control [20] . Allelic alterations of the Firre locus change Xi structure We evaluated chromatin accessibility in Firre mutants by ATAC-seq. As expected, in WT the distribution of allelic proportions centered at 0.5 for autosomes, but was skewed towards the Xa (0.95) for the X chromosomes, indicative of lower chromatin accessibility on the Xi. This pattern remained similar in Δ Firre Xa , consistent with near absence of gene reactivation. Plots of ATAC peak density further captured the low accessibility profiles of the Xi in both WT and Δ Firre Xa (Fig. 7a, b ). However, a higher peak density was observed in the telomeric region of the Xi in Δ Firre Xa where reactivated genes are located (Fig. 6c ; 7c ). ATAC-seq patterns were unchanged in Δ Firre Xi and Inv Firre Xi (Supplementary Fig. 6a, b ). To determine whether Dxz4 and Firre may have synergistic cis-effects on chromatin accessibility on the Xi, ATAC-seq was done on a double-mutant line Δ Firre Xi /Δ Dxz4 Xi . Interestingly, a pronounced shift to lower values in the distribution of allelic proportions for the X chromosomes (peak at ~0.55) was observed in this double-mutant compared to either Δ Dxz4 Xi (peak at ~0.85) or Δ Firre Xi (peak at ~1), indicating increased chromatin accessibility on the Xi (Fig. 7d, e ). Fig. 7: Chromatin accessibility after allelic Firre deletions and a Firre/Dxz4 deletion. a Density histograms of the distribution of allelic proportions ( spretus /( spretus + BL6)) of ATAC peaks along the autosomes and the X chromosomes for WT (blue) and Δ Firre Xa (red). No shift is observed (Wilcoxon test: −log10P = 32). b . Percentages of ATAC peaks along the autosomes and the X chromosomes classified as spretus -specific, BL6-specific, or both show no differences between WT (blue) and Δ Firre Xa (red). c . Plots of Xi-associated (common +Xi-specific) ATAC peak density (counts binned within 500 kb windows) along the Xi show increased accessibility at the telomeric end of the Xi in Δ Firre Xa (red) versus WT (blue). To account for differences in the number of SNP-covered peaks between samples due to sequencing depth, the binned counts are scaled by a factor obtained from the between-sample ratios of autosomal diploid SNP-covered peaks. d Density histograms of the distribution of allelic proportions ( spretus /( spretus + BL6)) of ATAC peaks show a shift to a lower Xa/(Xa + Xi) ratio in the double-mutant Δ Firre Xi /Δ Dxz4 Xi (purple), compared to Δ Dxz4 Xi (black) and Δ Firre Xi (green), consistent with increased accessibility on the Xi (Wilcoxon test: −log10P = 35). e Percentages of ATAC peaks in Δ Dxz4 Xi (black), Δ Firre Xi (green), and Δ Firre Xi /Δ Dxz4 Xi (purple) along the autosomes and the X chromosomes classified as spretus -specific, BL6-specific, or both show an increase on the BL6 Xi in the double mutant. Full size image Based on high-resolution allele-specific contact maps generated by DNase Hi-C the Xi bipartite structure was retained in Δ Firre Xi , but contacts increased between the superdomains and decreased within each superdomain, suggesting that the Firre locus acts in cis to help shape the 3D structure (Fig. 8a ). Contacts within regions flanked by Dxz4 and Xist (ChrX:75–100 Mb) and to a lesser extent, flanked by Firre and Dxz4 (ChrX:50–75 Mb) were increased, suggesting disruption of contacts emanating from Dxz4 (Fig. 8a , Supplementary Fig. 7a ). Similarly, Inv Firre Xi nuclei showed persistence of the Xi bipartite structure, but also a redistribution of contacts around Firre , including loss of proximal contacts (ChrX:5–50 Mb) and gain of distal contacts (ChrX:50–75 Mb), which was confirmed by virtual 4 C (Fig. 8a, b ; Supplementary Fig. 7a ). The boundary at or near the Firre locus on the WT Xi was maintained upon deletion or inversion of the locus (Supplementary Fig. 7b ). While the loss of Firre RNA in Δ Firre Xa did not perturb the bipartite structure of the Xi, there were some changes in contact distribution, suggesting trans-effects (Fig. 8c , Supplementary Fig. 7c ). Specifically, contacts increased in the region flanked by Dxz4 and Xist (ChrX:75–100 Mb), and diminished in the very distal telomeric region (ChrX:165–170 Mb), consistent with an increase in chromatin accessibility and gene expression (Figs. 6c , 7c , 8c ). Deletion of Firre on the Xa also resulted in contact changes on the Xa, including loss of the boundary at or close to the locus, as confirmed by insulation score analysis (Fig. 8d ; Supplementary Fig. 7d, e ). Fig. 8: Changes in the X 3D structure after Firre deletion or inversion. a Pearson correlated-transformed differential contact maps of the Xi at 500 kb resolution highlight differences between Δ Firre Xi and WT, and between Inv Firre Xi and WT. The color scale shows differential Pearson correlation values, with loss and gain of contacts in the mutants versus WT appearing blue and red, respectively. See text for description of changes. b Virtual 4 C plots derived from Hi-C data at 500 kb resolution using Firre as the viewpoint on the Xi in WT (blue), Δ Firre Xi (green) and Inv Firre Xi (gray) show an increase in contacts between Firre and Dxz4 in Inv Firre Xi . c Pearson correlated-transformed differential contact maps of the Xa and Xi at 500 kb resolution to highlight differences between Δ Firre Xa and WT. The color scale shows differential Pearson correlation values, with loss and gain of contacts in Δ Firre Xa versus WT appearing blue and red, respectively. See text for description of changes. d Pearson correlated-transformed contact maps (40 kb resolution) of the Xa for 4 Mb around the Firre locus highlight the loss of the strong boundary between TADs on the Xa in Δ Firre Xa versus WT (see Supplementary Fig. 7c for corresponding maps of the Xi). Full size image Taken together, our results indicate cooperation between Firre and Dxz4 in repression of chromatin accessibility on the Xi, with each locus contributing to the two superdomains separation. Firre contacts with other regions on the Xi appear orientation-dependent, reminiscent to the orientation-dependent contacts made by Dxz4 [29] . Firre RNA exerts trans-effects on the Xi 3D structure, potentially secondary to losses of H3K27me3 and CTCF binding. Studies of lncRNAs support the notion that these molecules can either spread in cis from their genomic locus or localize to cellular compartments away from their own locus of transcription to perform essential functions in regulating gene expression [52] , [53] , [54] , [55] . Here, we report that the lncRNA Firre transcribed from the Xa acts in trans and in cis on the Xi to maintain its epigenetic features, nuclear location, and 3D structure. LncRNAs have important roles in the structure of nuclei where they fold into higher-order structures and act in cooperation with proteins including chromatin-modifying complexes [56] . Xist represents the quintessential example of a lncRNA that spreads along the Xi in cis to recruit a series of proteins including components of the PRC complexes that implement chromatin modifications such as H3K27me3 [2] , [3] , [6] , [19] , [56] . We find that maintenance of H3K27me3 on the Xi mediated by Firre RNA involve the PRC complexes, which is supported by our reanalyses of RNA/protein interaction datasets [39] , [40] , [41] , [42] , [43] , [44] , [45] . Among Firre interactors EZH2 and SUZ12 represent core subunits of PRC2, while JARID2 and RBFOX2 are cofactors that directly interact with RNA [57] , [58] , [59] . PRC2 recruitment of the noncanonical PCGF3/5-PRC1 complex is facilitated by the Firre interactor hnRNPK [60] , while CBX7 is a subunit of the canonical PRC1 complex [61] . A new method to detect protein-RNA interactions (incPRINT) also identifies JARID2, EPC1, CTCF, and hnRNPU as Firre interactors [62] . Most Firre interactors have previously been implicated in XCI, and more specifically in H3K27me3 enrichment on the Xi (Supplementary Data 5 ) [2] , [6] , [63] , [64] , [65] , [66] . Colocalization of Firre RNA to the Xi was seen in only 15% of nuclei, suggesting dynamic binding of the lncRNA. Interestingly, single particle tracking of endogenous EZH2 and SUZ12 in human cells reveals rapid diffusion of PRC2 through the nucleus, with only ~20% chromatin-bound [67] . Trans-effects have been reported for several lncRNAs. For example, Fendrr and Pint recruit PRC2 for H3K27 tri-methylation of loci located on other chromosomes [68] , [69] . Meg3 also recruits PRC2 components, JARID2 and EZH2, to facilitate H3K27me3 deposition and repression of genes in trans [42] , [70] . Meg3 has an additional cis-acting role by sequestration of PRC2 to prevent DNA methylation-induced repression of genes within the Meg3-Mirg imprinting cluster [71] , [72] . Interestingly, we observe a local loss of H3K27me3 centering around the Firre locus and extending to 26 Mb in CLPs and CD8 + T cells from Firre KO female mice, suggesting that Firre may also act in cis to maintain H3K27me3 in certain cell types. Importantly, defects in hematopoiesis that impact CLPs have been observed in Firre KO mice [32] , [33] . Local cis-effects have also been demonstrated for the imprinted lncRNAs Airn and Kcnq1ot1 , which recruit the PRCs via hnRNPK to silence Mb-sized regions on one allele in cis [39] . Our results based on KD and transgenic rescue reveal dose-dependent effects of Firre RNA on H3K27me3 enrichment on the Xi, reminiscent of the dose-dependent silencing effects of Airn and Kcnq1ot1 [39] . The nucleolus has emerged as a platform for the organization of chromatin enriched in repressive histone modifications [16] , [17] , [18] , [73] . For example, loss of NPM1 results in deformed nucleoli and redistribution of H3K27me3 [74] . Depletion of Firre RNA limits association of the Xi to the nucleolus and nuclear periphery, supporting coordinated roles in Xi positioning and maintenance of H3K27me3 [20] . Two studies corroborate our findings: indeed, relocation of the Xi to the nucleolus during the cell cycle is required to maintain H3K27me3, and sparser H3K27me3 on the Xi occurs when it is kept away from the nucleolus or nuclear periphery [75] , [76] . Deletion of Xist also decreases both H3K27me3 enrichment and nucleolar association of the Xi [77] . However, we did not observe disruption of Xist RNA expression nor coating of the Xi in Δ Firre Xa nuclei, suggesting that Firre acts independently of Xist . On the other hand, CTCF, a protein that facilitates interactions between chromatin and the nucleolus may act in concert with Firre to help Xi positioning [51] . In addition to CTCF-DNA interactions CTCF-RNA interactions via specific zinc fingers represent important structural components of genome organization [78] . Such dual interactions characterize Firre since CTCF not only binds to the locus on the Xi, but also interacts with the RNA [20] , [21] , [62] . Thus, in the absence of Firre RNA disrupted Xi anchoring to the nucleolar periphery could result from the significant loss of CTCF binding observed along the entire Xi, including at the Firre locus. Supporting this notion, RNA depletion using RNase A disrupts the local chromatin environment around CTCF binding sites and the structural integrity of heterochromatin [38] . We cannot exclude other heterochromatin factors, for example, EZH1 or histone H1, both downregulated in Δ Firre Xa and rescued in transgenic lines [79] , [80] . Considering the 3D structure of the Xi, the Firre locus helps insulate the two superdomains of the Xi perhaps via CTCF binding and acts in synergy with Dxz4 to compact the Xi perhaps via a superloop with Dxz4 [27] . Our rescue experiments imply that a subset of Firre exons are sufficient for partial maintenance of H3K27me3 on the Xi and its location in the nucleus. It will be interesting to map additional functional units within the Firre locus, which may provide a more complete rescue. The Firre locus harbors several conserved local repeats and many of these do not overlap exons, except for the RRD repeats that display 65% identity between human and mouse, which makes them good candidates for the rescue function observed [21] , [23] . Notably, these repeats bind the nuclear matrix protein hnRNPU known to associate with Xist , the Xi, and other genomic regions [20] , [21] , [24] , [81] , [82] , [83] , [84] . 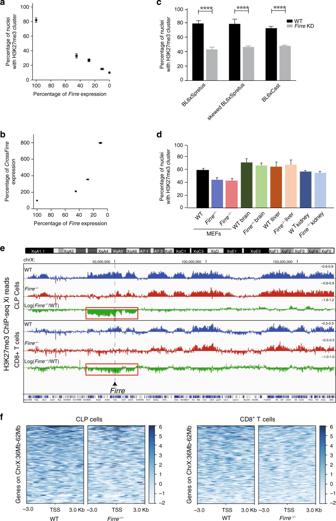Fig. 3: Dose-dependent effects ofFirreRNA on H3K27me3 on the Xi in cell lines and in vivo. aPercentage of nuclei with a H3K27me3 cluster after KD in Patski cells relative toFirreexpression level measured by qRT-PCR inn= 3 biologically independent samples. Data presented as mean values ± SEM.bThe level ofCrossFirreexpression is inversely related to that ofFirreafterFirreKD. Expression measured by qRT-PCR inn= 3 biologically independent samples. Data presented as mean values ± SEM.c, dA total of >300 Patski nuclei were scored per cell type over three independent experiments; significance was determined by one-sided Fisher exact test; bar plots are presented as mean values ± SEM; scale bars represent 10 µm.cBar plots show significantly fewer H3K27me3 clusters afterFirreKD in nuclei from three primary MEFs compared to mock treatment (pvalue = 2.89075e-12, 1.41519e-32, and 8.95838e-10, respectively). Primary MEFs were derived from a (BL6 ×spretus) embryo with aspretusXi, and from embryos either (BL6 ×spretus) or (BL6 ×castaneus) with random XCI (Table1).dBar plots show a lower (but not significantly) percentage of H3K27me3 cluster in nuclei from MEFs derived fromFirre+/−andFirre−/−KO embryos than in controls (pvalue = 0.0774 and 0.0567, respectively). No significant differences were found in brain, liver, and kidney fromFirreKO mice compared to WT (pvalue = 0.9127, 0.8796, and 0.762, respectively).eProfiles of H3K27me3 ChIP-seq reads along the X chromosomes from CLPs and CD8 + T cells from WT (blue),Firre−/−(red), and log2ratioFirre−/−/WT (green) show a significant decrease covering ~26 Mb around theFirrelocus in mutant CLPs, and to a lesser extent CD8 + T cells (Supplementary Data6).fHeatmaps of H3K27me3 ChIP-seq reads located 3 kb around the transcription start sites (TSS) of X-linked genes that map within the 26 Mb region aroundFirrein WT andFirre−/−CLPs and CD8 + T cells. Our findings of dysregulated genes implicated in cell cycle and development upon loss of Firre RNA support a role in cell growth, a common finding for other lncRNAs [85] . Both Firre KO mice and mice with Firre overexpression have abnormalities specifically in hematopoiesis, implying the importance of Firre dosage [32] , [33] . In human loss of FIRRE RNA causes dysregulation of inflammatory gene expression, while amplification of FIRRE causes congenital abnormalities and is associated with decreased survival rates in cancer, further supporting FIRRE dosage effects [24] , [85] , [86] . Despite ample evidence supporting their biological relevance in cell systems lncRNAs are often dispensable for survival of vertebrate organisms. For example, mice homozygous for deletions of regions harboring 1243 noncoding sequences had no distinguishable phenotypes [87] . Similarly, mice with deletions of nine conserved lncRNAs including Malat were viable with no obvious abnormalities [50] , [88] . Firre KO mice have few abnormal phenotypes except for abnormalities in B- and T-cell physiology [33] . This dearth of phenotypes could be explained by alternative pathways, possibly other lncRNAs that may compensate during development, providing redundancy in the system [89] . A recent publication reports that following 10 days of differentiation, mouse ES cells with a Firre deletion on the Xa, the Xi or on both alleles show no effects on H3K27me3 on the Xi, which differs from our results based on mutations induced in differentiated fibroblasts [35] . Thus, phenotypic effects apparently depend on the developmental timing of Firre mutations, and mutations at early stages may allow compensatory pathways to effectively help survival. Indeed, Firre KO ES cells display a marked decrease in growth rate, supporting the existence of critical mechanisms for survival of subsets of cells and subsequent differentiation/development [23] . In addition, differences in the effects of Firre mutations may reflect developmental stage-specific composition of PRC complexes [90] . Another important consideration is cell type specificity. There was no apparent loss of H3K27me3 on the Xi in brain, kidney, and liver from Firre KO mice. However, a local disruption of H3K27me3 around Firre was found in CLPs and CD8 + T cells, suggesting that Firre RNA may act in cis in certain cell types. In a CRISPRi phenotypic screen a majority of lncRNAs only displayed phenotypes in a single cell type [50] . A new approach, PIRCh-seq, designed to find association between RNA and specific chromatin modifications reports Firre interactions with H3K27me3 chromatin in MEFs, but not in ES cells, highlighting differences between cell types [91] . Furthermore, mouse and human Firre / FIRRE exhibit diverse expression patterns across tissues, e.g., enrichment in neural crest but depletion in lung fibroblasts [23] . Firre KO mice show organ-dependent gene dysregulation, with a larger number of dysregulated genes in spleen, which can be rescued by ectopic Firre expression supporting a trans-acting role in vivo [32] , [33] . The gene expression changes we observed in kidney-derived Patski cells differ from those reported in Firre KO mouse spleen, again suggesting tissue-specificity. In immune cells where Firre RNA exerts a local cis-effect on the Xi, it remains to be determined whether Firre might be expressed from the Xi. Interestingly, female lymphocytes lack Xist clouds and H3K27me3 foci, and show reactivation of the Xi [92] . Further analyses to distinguish alleles is needed to better understand Firre local effects in immune cells. Cell lines The Patski cell line, originally derived from embryonic kidney (18.5 dpc) from a cross between a female C57BL/6 J (BL6) with an Hprt BM3 mutation and a male Mus spretus ( spretus ), was previously selected in HAT (hypoxanthine-aminopterin-thymidine) medium so that the Xi is always from BL6 [93] , [94] . Primary MEF cultures were derived from a 13.5 dpc female embryo resulting from a BL6 × Mus spretus cross, which results in skewed inactivation of the spretus X chromosome due to an Xist mutation on the BL6 X chromosome [95] . Primary MEFs were also derived from BL6 × Mus spretus and BL6 × Mus castaneus 13.5 dpc female F1 embryos with random XCI. Cells were cultured as described and the presence of normal X chromosomes verified by karyotyping [29] . For ectopic Firre expression assays in Patski cells and in MEFs, a mouse Firre cDNA plasmid (mtransgene; Dharmacon BC055934) or a human FIRRE cDNA plasmid (htransgene; Dharmacon BC038558) were each transfected together with the selectable marker pPGK-Puro plasmid (gift from R. Jaenisch; Addgene 11349) into Δ Firre Xa cells using lipofectamine 3000 (Invitrogen). Blast searches were performed to map homology of the cDNAs to the reference genomes (Supplementary Fig. 1b ). After transfection, Δ Firre Xa+mtransgene and Δ Firre Xa+htransgene were selected in Eagle’s medium with 2 µg/ml puromycin for 72 h, followed by recovery in Eagle’s medium with 1 µg/ml puromycin for 10 days. A Δ Firre Xa+mtransgene clone with high Firre expression was also isolated. KO mouse tissues and isolation of CLPs and CD8 + T cells Mice used in this study were maintained in pathogen-specific-free facilities under the supervision of either the University of Washington Institutional Animal Care and Use Committee (Protocol number 2254) or Harvard University’s Institutional Animal Care Committee. We complied with the ethical regulations for animal testing and research in accordance with these committees. Tissues collected from a Firre KO mouse model included liver, kidney, and brain from heterozygous ( Firre +/− ) and homozygous ( Firre −/– ) mutants, and from control female mice verified by genotyping [33] . Ectopic expression of Firre induced by doxycycline (DOX) injection in mice was done as described [33] . 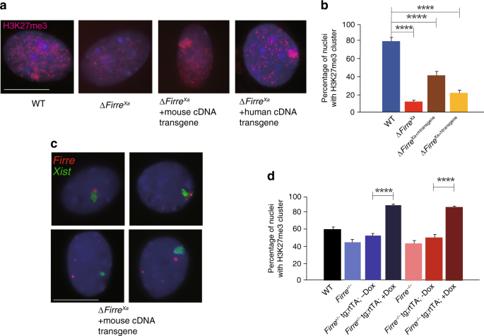Fig. 4: Ectopic expression ofFirre/FIRRERNA partially restore H3K27me3 on the Xi. aExamples of nuclei after H3K27me3 immunostaining (red) and Hoechst 33342 staining (blue) in WT, ΔFirreXa, and ΔFirreXatransfected with a mouseFirretransgene (ΔFirreXa+mtransgene) or a humanFIRREtransgene (ΔFirreXa+htransgene).bThe bar plot shows a significantly higher percentage of nuclei with a H3K27me3 cluster in cells with a mouse or humanFirre/FIRREtransgene, compared to ΔFirreXa(pvalue = 2.8075e-16 and 0.0000134599, respectively).cExamples of nuclei after RNA-FISH forXist(green) andFirre(red) in a ΔFirreXa+mtransgenecell clone with high expression of the mouse transgene. The upper two nuclei show association betweenFirreandXistsignals (seen in 15% of nuclei), and the lower nuclei, lack of association.dThe bar plot shows the percentage of nuclei with a H3K27me3 cluster in MEFs derived fromFirre+/−andFirre−/−females that harbor a doxycycline (Dox) inducible transgene (Firre+/−tg;rtTA; -Dox;Firre+/−tg;rtTA; +Dox;Firre−/−tg;rtTA; -Dox;Firre−/−tg;rtTA; +Dox), compared to WT and mutants. The percentage of nuclei with a H3K27me3 cluster increases significantly inFirre+/−tg;rtTA andFirre−/−tg;rtTA MEFs after addition of doxycycline (Dox+) (p value=4.31567e-30 and 3.51193e-20, respectively). A total of >300 nuclei scored for the presence of a H3K27me3 cluster (a,b, d), or forXistandFirreRNA-FISH signals (c) per cell type over three independent experiments; significance was determined by one-sided Fisher exact test; bar plots are presented as mean values ± SEM; scale bars represent 10 µm. MEFs were derived from mutant ( Firre +/− , Firre −/− ) and control female 13.5 dpc embryos. We isolated CLPs live [Lin–Sca-1locKitloIL7Rα+] by fluorescence-activated cell sorting (FACS) from WT (age: 35–43 days) and Firre −/− (age: 35 days) female mice to generate two replicate samples per genotype, consisting of two mice per replicate. Bone marrow was isolated from both femurs and tibias of each mouse by removing the end caps and flushing the bone marrow with a 27 G syringe containing staining media (DMEM, Gibco, 11995–073) with 5% fetal bovine serum (FBS, Gibco, 26140079) and 10 mM EDTA into a 50 mL conical tube. Cells pelleted by centrifugation at 1200 rpm were subjected to lineage depletion according to the manufacturer’s protocol (Miltenyi Biotec, 130–090–858). Lineage-depleted bone marrow was resuspended with the following antibodies (1:100): PE/Cy7 anti-mouse CD127 (IL-7Rα) clone A7R34 (Biolegend, 135014), Alexa Fluor 488 anti-mouse CD117 (c-Kit) clone 2B8 (Biolegend, 105816), PE/Dazzle-594 anti-mouse Ly-6A/E (Sca-1) clone D7 (Biolegend, 108138), APC anti-mouse CD34 clone HM34 (Biolegend, 128612), PE anti-mouse CD135 clone A2F10 (Biolegend, 135306), and Pacific Blue anti-mouse Lineage Cocktail (20 μL per 1 × 106 cells) clones 17A2/RB6-8C5/RA3-6B2/Ter-119/M1/70 (Biolegend, 133310). Zombie Aqua Fixable Viability Kit (Biolegend, 423101) was used as a viability stain according to the manufacturer’s protocol. Samples were incubated on ice in the dark for 60 min, washed twice with staining media, and resuspended before sorting by FACS (BD Aria). To isolate CD8 + T-cells peripheral blood was collected from mice by cardiac puncture into a tube containing 4% citrate. Red blood cells were lysed for 15 min at room temperature using BD Pharm Lyse (BD, 555899). Cells were washed twice with staining media and the following antibodies were added (1:100) to each sample prior to incubation for 30 min at room temperature: PE anti-mouse CD3 clone 17A2 (Biolegend, 100205), Alexa Fluor 700 anti-mouse CD8a clone 53–6.7 (Biolegend, 100730), APC anti-mouse CD19 clone 6D5 (Biolegend, 115512), Alexa Fluor 488 anti-mouse NK-1.1 clone PK136 (Biolegend, 108718), PE/Dazzle-594 anti-mouse CD4 clone GK1.5 (Biolegend, 100456), TruStain FcX (anti-mouse CD16/32) clone 93 (1:50) (Biolegend, 101319). Zombie Aqua Fixable Viability Kit (Biolegend, 423101) was used as a viability stain. Cells were washed twice with staining media and sorted by FACS (BD Aria). Allele-specific CRISPR/Cas9 editing and RNAi KD For allele-specific CRISPR/Cas9 editing of the endogenous Firre locus, three highly specific sgRNAs with BL6 or spretus SNPs at the PAM site and with low off-target scores were chosen and aligned back to the reference genome using BLAT (UCSC) to verify specificity (Supplementary Data 1 ). The sgRNAs cloned into p × 330 plasmids (Addgene) were transfected into WT Patski cells using Ultracruz reagents (Santa Cruz). A Patski line with a deletion of Dxz4 was also transfected to generate a double-mutant Δ Firre Xi /Δ Dxz4 Xi [29] . Single-cell derived colonies were selected and deletions or inversions of the targeted Firre locus verified using PCR and Sanger sequencing to confirm allele-specific editing (Supplementary Data 2 ). Firre RNAi KD was performed as described [20] . Cells were harvested after double shRNA/siRNA treatment and qRT-PCR performed to verify KD efficiency. Immunofluorescence, RNA-FISH, and DNA-FISH Immunofluorescence was done on cells grown on chamber slides, fixed with paraformaldehyde, permeabilized, and blocked as described previously [20] . Mouse liver, kidney, and brain were embedded in a cassette and sectioned by the University of Washington histopathology service center. Tissue sections (5 µm) were permeabilized using 0.5% Triton X-100 for 10 min and fixed in 4% paraformaldehyde for 10 min. After incubation with a primary antibody specific for H3K27me3 (Upstate/Millipore, #07–449), H2AK119ubi (Cell Signaling, #8240 S), macroH2A (Abcam, #ab37264), or NPM1 (Abcam, #ab10530) overnight at 4 °C in a humidified chamber cells/tissue sections were washed in 1× PBS (phosphate-buffered saline) buffer and incubated with a secondary antibody conjugated to Texas Red (anti-rabbit, Vector, # TI-1000) or fluorescein (anti-mouse, Vector, # FI-2100). RNA-FISH for Xist was done using a labeled 10 kb cDNA plasmid (pXho, which contains most of Xist exon 1) as described [20] . RNA-FISH for Firre was done in a clonal Δ Firre Xa+mtransgene line that overexpresses Firre RNA using a labeled plasmid probe containing Firre cDNA. DNA-FISH was done using labeled BAC probes containing Firre (RP24-322N20) or Dxz4 (RP23-299L1) [29] . Images were acquired with a Zeiss fluorescence microscope equipped with an image capture system ZEN 2.3. Slides were examined by fluorescence microscopy to score the number of nuclei with enrichment in each histone modification on the Xi, using Xist RNA-FISH for Xi identification. A minimum of 300 nuclei were scored per cell type by at least two observers. Measurements of overall H3K27me3 staining intensity outside the Xi cluster were done in a minimum of 300 nuclei using ImageJ [36] . To minimize experimental variance, a mixture of 80% Δ Firre Xa and 20% WT cells were grown in the same chamber prior to immunostaining with H3K27me3 and a control histone panH4 (Abcam ab10158), together with DNA counterstaining using Hoechst 33342. Selected nuclear areas away from the Xi were used for measurement of H3K27me3 median intensity, with same-area normalization to either Hoechst 33342 or panH4 staining. Comparisons between WT and Δ Firre Xa were done by calculating either the H3K27me3 staining intensity versus Hoechst 33342 and panH4 for WT and Δ Firre Xa nuclei separately, or the relative H3K27me3 staining intensity in Δ Firre Xa versus WT nuclei present in the same microscope field. The location of the Xi with respect to the nuclear periphery and the edge of the nucleolus (labeled with NPM1) was recorded in at least 300 nuclei. Allelic in situ Hi-C, CUT&RUN, ATAC-, RNA-, and ChIP-seq In situ DNase Hi-C was done on intact nuclei from Δ Firre Xa , Δ Firre Xi , Inv Firre Xi , and WT as described [29] , [30] . Hi-C libraries were sequenced using 150 bp paired-end reads (Supplementary Data 11 ). ATAC-seq on Δ Firre Xa , Δ Firre Xi , Inv Firre Xi , Δ Firre Xi /Δ Dxz4 Xi , and WT, and RNA-seq on Δ Firre Xa , Δ Firre Xa+mtransgene , and WT were done as previously described [29] . ChIP-seq was done on Δ Firre Xa and WT using an antibody for H3K27me3 and an established protocol [20] . CUT&RUN was done on Δ Firre Xa , Δ Firre Xa+mtransgene , and WT using an antibody for CTCF (Upstate/Millipore, 07-729-25UL), and on Δ Firre Xa and WT using an antibody for SUZ12 (Abcam ab12073) using a published protocol [96] . H3K27me3 ChIP analyses of CLPs and CD8 + T cells were done using the TrueMicroChIP kit (Diagenode, C01010130) according to the manufacturer’s protocol. Briefly, we sheared fixed chromatin from ~32,000 CLPs and ~50,000 CD8 + T cells in separate 1.5 mL TPX plastic tubes (Diagenode, C3001001050) using the following cycles on a Bioruptor (Diagenode): eight cycles of 5 min (30 ON, 30 OFF). Between each cycle samples were placed on ice. Sheared chromatin was then immunoprecipitated using 1 µL of H3K27me3 antibody (Diagenode, C15410069), retaining 10% of the chromatin as input. ChIP products were eluted in 12 µL and libraries prepared using the MicroPlex Library Preparation kit v2 (Diagenode, C05010012). Ten microleter of ChIP products were used as input, iPCRtagT1-T12 were used for 12 amplification cycles. After library clean up, the libraries were analyzed on a BioAnalyzer DNA-HS chip. 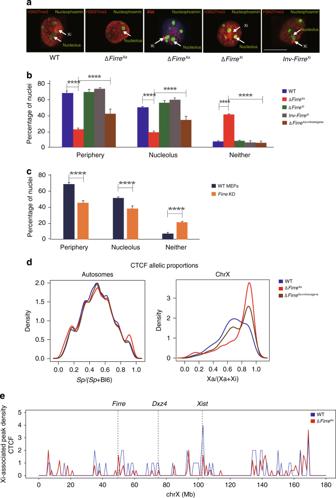Fig. 5:FirreRNA acts in trans to maintain Xi location. a–cA total of >300 nuclei per cell type over 3 independent experiments were scored for the location of the Xi marked by a H3K27me3 cluster or anXistcloud relative to the nuclear periphery or the nucleolus; significance was determined by one-sided Fisher exact test; bar plots are presented as mean values ± SEM; scale bars represent 10 µm.aExamples of nuclei after H3K27me3 immunostaining (red) to locate the Xi in WT, ΔFirreXi, and InvFirreXi, orXistRNA-FISH (red) to locate the Xi in ΔFirreXasince there is no H3K27me3 cluster in these nuclei. Nuclei were also immunostained for NPM1 (green) to locate the nucleolus.bBar plots show a significant decrease in periphery- and nucleolus association of the Xi in ΔFirreXacompared to WT (pvalue = 3.95632e-40 and 3.75497e-14, respectively), but no significant changes in ΔFirreXiand InvFirreXi(pvalue = 0.6968). Ectopic expression of a mouse transgene in ΔFirreXa+mtransgenepartly rescues the Xi location to 41% at the periphery and 34% at the nucleolus (pvalue = 6.62701e-10 and 0.000265481, respectively).cBar plots show a significant decrease in periphery- and nucleolus association of the Xi afterFirreKD in primary MEFs derived from an F1 embryo (BL6 ×spretus) (pvalue = 1.13757e-09 and 0.0000634923, respectively).dDensity histograms of the distribution of allelic proportions (Xa/(Xa + Xi)) of CTCF peaks show a shift in the distribution for the X chromosomes due to a decrease in CTCF on the Xi in ΔFirreXa(red) compared to WT (blue). In ΔFirreXa+mtransgene(brown) this distribution becomes binomial due to partial restoration of CTCF on the Xi.ePlots of Xi-associated (common +Xi-specific) CTCF peak density (counts binned within 100 kb windows) along the Xi for WT (blue) and ΔFirreXa(red). To account for differences in the number of SNP-covered peaks due to sequencing depth, the binned counts are scaled by a factor obtained from the between-sample ratios of autosomal diploid SNP-covered peaks. ATAC-seq, ChIP-seq, and CUT&RUN libraries for Patski cells were sequenced as 75 bp pair-end reads (Supplementary Data 11 ). RNA-seq libraries for Patski cells were sequenced as 75 bp single-end reads (Supplementary Data 11 ). Sequencing datasets were analyzed to assign reads to the spretus or BL6 genomes using a previously developed allele-specific data analysis pipeline [29] . RNA-seq reads were mapped to the UCSC mm10 (NCBI build v38) refSeq BL6 mouse transcriptome. Tophat2 (v 2.0.12) (calling bowtie2 (v2.2.3)) was used to perform single-end mapping allowing six mismatches. Mapped reads were assigned to refSeq genes using HT-seq(v0.11.0) and counts were converted into TPMs using custom R scripts. DE analysis was performed using DESeq2. 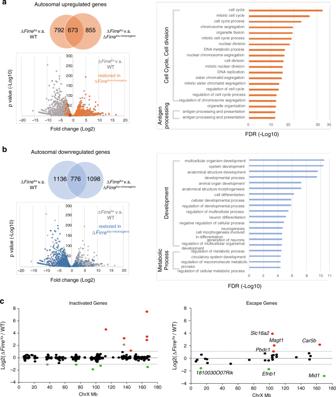Fig. 6: Loss ofFirreRNA affects gene expression. aUpregulated genes in ΔFirreXaand Gene Ontology (GO) term enrichment. The Venn diagram shows the number of upregulated genes in ΔFirreXaversus WT, and in ΔFirreXaversus ΔFirreXa+mtransgene, with the overlapping gene set representing upregulated genes in ΔFirreXathat are rescued by transgene expression. The scatter plot shows dysregulated genes in ΔFirreXaversus WT (grey), with genes rescued by reduced expression in ΔFirreXa+mtransgeneversus ΔFirreXa(more than 2-fold;pvalue < 0.05 by the Wald test) highlighted in orange. The top 20 GO terms of overlapping upregulated genes in ΔFirreXaversus WT, which are rescued in ΔFirreXa+mtransgeneare listed. TheX-axis indicates the FDR (−log10).bDownregulated genes in ΔFirreXaand Gene Ontology (GO) term enrichment. The Venn diagram shows the number of downregulated genes in ΔFirreXaversus WT, and in ΔFirreXaversus ΔFirreXa+mtransgene, the overlapping gene set representing downregulated genes in ΔFirreXathat are rescued by transgene expression. The scatter plot shows dysregulated genes in ΔFirreXaversus WT (gray), with genes rescued by increased expression in ΔFirreXa+mtransgeneversus ΔFirreXa(more than 2-fold;pvalue <0.05 by the Wald test) highlighted in blue. The top 20 GO terms of overlapping downregulated genes in ΔFirreXaversus WT, which are rescued in ΔFirreXa+mtransgeneare listed. TheX-axis indicates the FDR (−log10).cXi-expression fold changes for genes that are subject to or escape XCI between ΔFirreXaand WT. Upregulated genes are in red and downregulated genes in green. To note, one upregulated gene and one gene subject to XCI are in gray, as they showed more than 2-fold change in expression but with apvalue >0.05 by the Wald test in ΔFirreXaversus WT. Genes are ordered from centromere to telomere along the Xi. ATAC-seq, ChIP-seq, and CUT&RUN reads were mapped to the BL6 mouse genome using the NCBI build v38/mm10 reference genome assembly obtained from the UCSC Genome Browser using BWA-MEM (v0.7.3) in paired-end mode using default parameters. Peaks were called using MACS2. DNase Hi-C reads were mapped to the BL6 genome using the NCBI build v38/mm10 reference genome assembly obtained from the UCSC Genome Browser and a pseudo-spretus genome using BWA-MEM (v0.7.3) in single-end mode using default parameters [29] . Micro-RNA-seq (less than 200nt) was done in Δ Firre Xa and WT Patski cells by BGI Genomics ( https://www.bgi.com/us/ ). 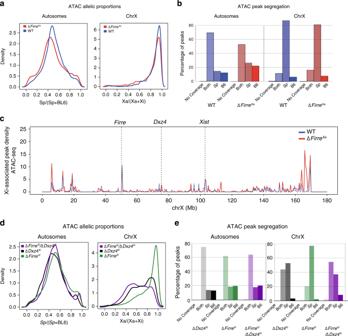Fig. 7: Chromatin accessibility after allelicFirredeletions and aFirre/Dxz4deletion. aDensity histograms of the distribution of allelic proportions (spretus/(spretus+ BL6)) of ATAC peaks along the autosomes and the X chromosomes for WT (blue) and ΔFirreXa(red). No shift is observed (Wilcoxon test: −log10P = 32).b. Percentages of ATAC peaks along the autosomes and the X chromosomes classified asspretus-specific, BL6-specific, or both show no differences between WT (blue) and ΔFirreXa(red).c. Plots of Xi-associated (common +Xi-specific) ATAC peak density (counts binned within 500 kb windows) along the Xi show increased accessibility at the telomeric end of the Xi in ΔFirreXa(red) versus WT (blue). To account for differences in the number of SNP-covered peaks between samples due to sequencing depth, the binned counts are scaled by a factor obtained from the between-sample ratios of autosomal diploid SNP-covered peaks.dDensity histograms of the distribution of allelic proportions (spretus/(spretus+ BL6)) of ATAC peaks show a shift to a lower Xa/(Xa + Xi) ratio in the double-mutant ΔFirreXi/ΔDxz4Xi(purple), compared to ΔDxz4Xi(black) and ΔFirreXi(green), consistent with increased accessibility on the Xi (Wilcoxon test: −log10P = 35).ePercentages of ATAC peaks in ΔDxz4Xi(black), ΔFirreXi(green), and ΔFirreXi/ΔDxz4Xi(purple) along the autosomes and the X chromosomes classified asspretus-specific, BL6-specific, or both show an increase on the BL6 Xi in the double mutant. 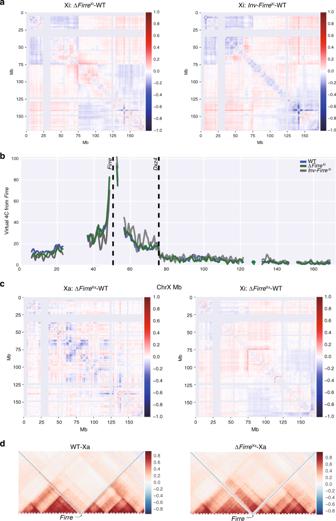Fig. 8: Changes in the X 3D structure afterFirredeletion or inversion. aPearson correlated-transformed differential contact maps of the Xi at 500 kb resolution highlight differences between ΔFirreXiand WT, and between InvFirreXiand WT. The color scale shows differential Pearson correlation values, with loss and gain of contacts in the mutants versus WT appearing blue and red, respectively. See text for description of changes.bVirtual 4 C plots derived from Hi-C data at 500 kb resolution usingFirreas the viewpoint on the Xi in WT (blue), ΔFirreXi(green) and InvFirreXi(gray) show an increase in contacts betweenFirreandDxz4in InvFirreXi.cPearson correlated-transformed differential contact maps of the Xa and Xi at 500 kb resolution to highlight differences between ΔFirreXaand WT. The color scale shows differential Pearson correlation values, with loss and gain of contacts in ΔFirreXaversus WT appearing blue and red, respectively. See text for description of changes.dPearson correlated-transformed contact maps (40 kb resolution) of the Xa for 4 Mb around theFirrelocus highlight the loss of the strong boundary between TADs on the Xa in ΔFirreXaversus WT (see Supplementary Fig.7cfor corresponding maps of the Xi). ChIP-seq libraries for CLPs and CD8 + T cells were sequenced as 150 bp pair-end reads. Sequencing datasets were analyzed to assign reads to the BL6 genome using the NCBI build v38/mm10 reference genome assembly obtained from the UCSC Genome Browser using Bowtie2. Differential tracks and heatmaps were generated by Deeptools. GO analysis was done using http://geneontology.org/ .